Palladium-catalysed formation of vicinal all-carbon quaternary centres via propargylation Construction of two vicinal all-carbon quaternary carbon centres is of great importance due to the common presence of such units in natural and unnatural molecules with attractive functions. However, it remains a significant challenge. Here, we have developed a palladium-catalysed general coupling for the efficient connection of two tertiary carbon atoms: Specifically, propargylic carbonate has been treated with a fully loaded soft functionalized nucleophile to connect such two fully loaded carbon atoms with a simple palladium catalyst. It is observed that the central chirality in the optically active tertiary propargylic carbonates has been remembered and transferred into the products with very high efficiency. The triple bond and the functional groups such as ester, cyano and unsaturated C–C bonds make this method a relatively general solution for such a purpose due to their high synthetic versatility. Carbon-carbon bond formation is an ever-lasting topic in organic chemistry-related sciences such as synthesis, drug discovery and materials. Of particular interest is a contiguous array of all-carbon quaternary centres, which are found in many complex natural products with remarkable biological activities [1] , [2] , [3] , [4] . However, the efficient creation of such entities by carbon-carbon bond formation reaction is still challenging [5] , [6] , [7] . The most direct approach would be the coupling reaction of two related carbon species; however, this is largely underdeveloped due to the extremely strong steric effect and the intrinsic challenge of β-H elimination forming the olefins (equations (1) and (2), Fig. 1a ). For a selection of such efforts, see refs 8 , 9 , 10 , 11 . So far, the commonly notable approach is the allylic substitution reaction with an issue of regioselectivity, which is obviously still in its early stage in terms of the scope (equation (3), Fig. 1a ) [12] , [13] , [14] , [15] , [16] , [17] , [18] , [19] . 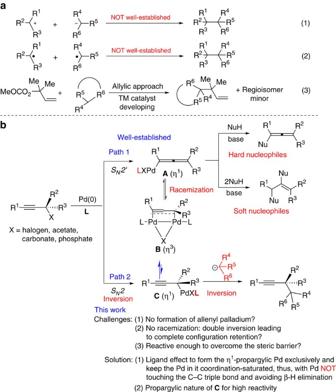Figure 1: Formation of vicinal all-carbon quaternary centres. (a) Previous works. (b) This work: new concept for vicinal all-carbon quaternary centres. Figure 1: Formation of vicinal all-carbon quaternary centres. ( a ) Previous works. ( b ) This work: new concept for vicinal all-carbon quaternary centres. Full size image Propargylic carbonates are a class of very common organic compounds with already well-established versatile attractive reactivities in organic synthesis. Since Tsuji’s first report in 1985 (ref. 20 ), palladium-catalysed transformations of propargylic alcohols or their derivatives have become a useful tool for constructing carbon–carbon and carbon–heteroatom bonds. In most cases, these reactions give rise to the corresponding allenyl palladium species A via different approaches ( S N 2 ′-type oxidative addition plus S N 2 -type oxidative addition followed by isomerization via intermediate B ), which was followed by the coupling reaction with a hard carbon nucleophile to form the allene derivatives or by the attack of two molecules of soft carbon nucleophiles to form the corresponding alkene derivatives (Path 1, Fig. 1b ) [21] , [22] . In rare cases, the direct propargylic substitution with simple carbon nucleophiles has been reported as the minor byproducts or major products (Path 2, Fig. 1b ) [23] , [24] , [25] , [26] , [27] ; however, to the best of our knowledge, the propargylations of tertiary propargylic alcohol derivatives with fully loaded soft carbon nucleophiles have never been realized. We reasoned that, by applying a suitable ligand together with optimized reaction parameters, the S N 2 ′-type oxidative addition would be shut down; with that the S N 2 -type oxidative addition would give η 1 -propargylic palladium C exclusively with the absolute configuration inverted. If such a ligand makes the palladium in C coordination-saturated, this intermediate would NOT isomerize to η 1 -allenylic palladium A mostly via the intermediacy of η 3 -dinuclear palladium intermediate B , as shown by Ogoshi et al . [28] . In addition, the intrinsic β-H elimination should also be avoided for the same reason. Finally, the highly reactive propargylic nature may make this intermediate C reactive enough to undergo reaction with a sterically hindered tertiary carbon nucleophile. If the stereoselectivity may be controlled, an efficient, highly stereoselective connection of two tertiary carbon atoms may be fulfilled. As an extra bonus, the synthetic potential of the C–C triple bond is attractive, since it may undergo further deliberate synthetic elaboration for different purposes as compared with the allylic approach shown in equation (3) of Fig. 1a . In this paper, we wish to report our recent realization of such a concept: the palladium-catalysed reaction of tertiary propargylic carbonates with different fully-loaded carbon nucleophiles to form such carbon–carbon bonds, which nicely remembers the central chirality in the starting propargylic carbonates by applying dppf as the proper ligand. Optimization of the reaction Initially we were studying the coupling cyclization reactions of 2-(2,3-butadienyl)malonitrile 2a with propargylic carbonate 1a for the synthesis of allene compounds 5aa and 6aa (ref. 29 ). After many trial and error methods with different ligands, Pd catalysts and other reaction parameters, we failed to observe the formation of the expected products 5aa and 6aa from the reaction of methyl (2-methyl-4-phenylbut-3-yn-2-yl) carbonate 1a (0.3 mmol) with 2-(buta-2,3-dien-1-yl)malononitrile 2a (1.5 equiv.) under the catalysis of Pd(OAc) 2 (5 mol%) and a ligand (6 mol%) with K 2 CO 3 (3.0 equiv.) at 30 °C in dimethylsulphoxide (DMSO) for 6 h (entries 1–7, Table 1 ). However, when we used dppe, dppb and BINAP as the ligand, surprisingly, the reaction afforded the targeted propargylic substitution product 3aa in Fig. 1 with two continuous carbon centres, albeit in very low yields, exclusively (entries 2, 4 and 5, Table 1 ). Encouraged by this exciting discovery of the formation of two vicinal all-carbon quaternary centres, the influence of the critical reaction parameters was investigated and it was found that 3aa was formed in 94% isolated yield by running the reaction with dppf, a very bulky ligand (entry 8, Table 1 )! After screening a series of solvents, DMSO was still proved to be the best: the reactions in tetrahydrofuran, CH 3 CN, dimethylformamide or dimethylacetamide all afforded lower yields of 3aa with some recovery of 1a (entries 11–14, Table 1 ). Thus, the conditions presented in entry 8 of Table 1 have been chosen as the standard for further study. Table 1 Optimization of reaction conditions*. Full size table Substrate scope With the optimized conditions in hand (entry 8, Table 1 ), we first examined the reactivity of various tertiary propargylic carbonates 1 with 2-(buta-2,3-dien-1-yl)malononitrile 2a . The substrates with the R 1 substituent of the alkyne unit being aryl bearing either electron-deficient or electron-rich groups could all proceed smoothly, affording the expected 1,6-allenyne products in 85–90% yields ( 3aa – 3da ); moreover, the method could be extended to 3-thienyl or n -Bu-substituted propargylic carbonates in 84% yield ( 3ea , 3fa ). In addition, the carbonates where R 2 , R 3 bore different groups could also be introduced into this transformation in good yields ( 3ga – 3ia ). It is worthy of mention that the reaction afforded the corresponding products 3ja and 3ka in moderate yields when cyclic tertiary propargylic carbonates 1j and 1k (see Supplementary Information for the structures) were applied. The practicality of this reaction has been demonstrated by running the reaction of 1a on a 10 mmol scale ( 3aa ) and 1j on an 8.4 mmol scale ( 3ja ). We next explored the scope of functionalized tertiary carbon nucleophiles under optimized conditions. For the 2,3-allenyl malononitriles, we could introduce the n -pentyl group at the 2-position ( 3lb ) or the Cy group at the 4-position ( 3mc ); to our delight, different propargylic malononitriles could be applicable to this reaction, affording the 1,6-diyne products in 84–92% yields ( 3ad – 3of ); when various allyl malononitriles were used, the 1,6-enyne products were obtained in excellent yields ( 3ag – 3pi ); we also prepared the 1,5-diphenylhexyne derivatives 3aj in 94% yield and 3gj in 92% yield with 2-benzylmalononitrile used as the nucleophile. In addition, the method is also proper to a C 10 -alkyl-substituted malononitrile ( 3ak ). Besides the malononitriles, the tertiary carbon nucleophiles could also be substituted methyl 2-cyanoacetates ( 3al – 3an ) and dimethyl malonate ( 3ao and 3ap ). 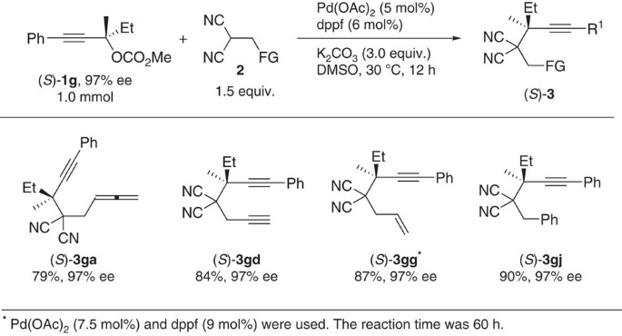Figure 2: Highly entioselective synthesis by chirality transfer. Excellent efficiency of chirality transfer was found when using (S)-1g. Table 2 The scope of the tertiary propargylic carbonates and tri-substituted carbon nucleophiles* † ‡ § || . Full size table In order to unveil the mechanism ( Fig. 4 ), the reactions of ( S )- 1g (refs 30 , 31 ) (97% ee), which has a chiral quaternary carbon centre, with different functionalized malononitriles were tried. To our surprise, all the corresponding products, ( S )- 3ga , ( S )- 3gd , ( S )- 3gg and ( S )- 3gj , were formed with the absolute configuration of the propargylic carbon atom remaining intact and with essentially no loss of enantiomeric purity ( Fig. 2 ). Figure 2: Highly entioselective synthesis by chirality transfer. Excellent efficiency of chirality transfer was found when using ( S )- 1g . 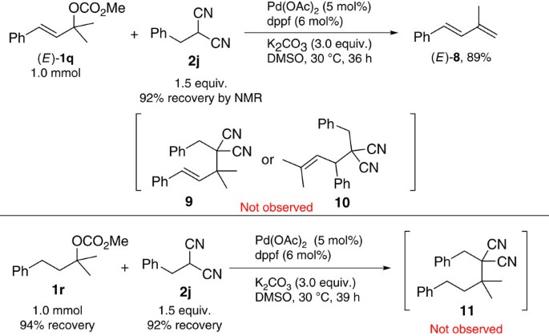Figure 3: The unique role of the carbon–carbon triple bond. (E)-1qand1rfailed to afford the corresponding vicinal all-carbon quaternary centres. Full size image Figure 3: The unique role of the carbon–carbon triple bond. ( E )- 1q and 1r failed to afford the corresponding vicinal all-carbon quaternary centres. 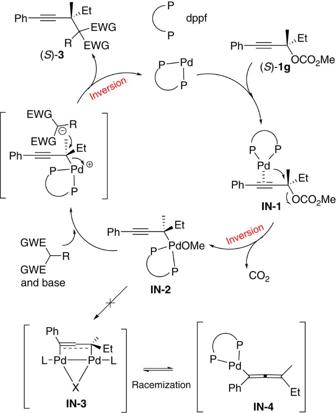Figure 4: A plausible mechanism. Dppf helps to keep the tetra-dentated palladium coordination saturated avoiding racemization. Full size image Figure 4: A plausible mechanism. Dppf helps to keep the tetra-dentated palladium coordination saturated avoiding racemization. Full size image In order to demonstrate the role of the unique carbon–carbon triple bond, some control experiments were conducted: (1) the reaction of tertiary allylic carbonate ( E )- 1q with 2-benzylmalononitrile 2j under the standard conditions failed to afford the expected allyl nucleophilic product 9 or 10 . Instead, the β-elimination product, that is, conjugated diene ( E )- 8 , was afforded in 89% yield. (2) On replacing carbonate ( E )- 1q with saturated tertiary carbonate 1r , no reaction occurred ( Fig. 3 ). Thus, it is concluded that the carbon–carbon triple bond in 1 plays a unique role in this nucleophilic substitution reaction. Based on these results, we propose a possible mechanism, as shown in Fig. 4 . The coordination of the C–C triple bond in ( S )- 1g with Pd(0) leads to the formation of coordination complex IN-1 . Oxidative addition of the chiral tertiary propargylic carbonate ( S )- 1g with Pd(0) would afford the propargyl η 1 -palladium intermediate IN-2 with the first inversion of the absolute configuration of the propargylic carbon atom. Dppf helps to keep this tetra-dentated palladium without forming η 3 -dinuclear palladium intermediate IN-3 , which avoids any possible racemization through the σ–π–σ isomerization process [28] . Subsequently, the in-situ -generated soft carbon nucleophile would attack this chiral carbon atom from the back side of the C–Pd bond to afford the final nucleophilic substitution product ( S )- 3 with the absolute configuration inverted for the second time and the regeneration of the catalytically active Pd(0). Overall, the absolute configuration of this propargylic carbon atom remains NOT inverted. Of course, the complete exclusion of allenyl palladium intermediate IN-3 is NOT possible, although such an option may most likely lead to at least partial racemization (see also Fig. 2 ) [32] . Such propargylation products have been demonstrated to be very useful in synthesis of different molecules with two continuous all-carbon quaternary carbon centres in high efficiency, as shown in Fig. 5 : (1) Tricyclic 1 H -cyclopenta[ b ]naphthalene derivative ( S )- 12 was prepared from a tandem reaction of ( S )- 3gd and 1-iodo-4-nitrobenzene [33] . In fact, the absolute configuration of the chiral propargylation products ( S )- 3ga , ( S )- 3gd , ( S )- 3gg and ( S )- 3gj has been established on the basis of an X-ray single-crystal diffraction study of this product. (2) The 1,6-allenyne derivative 3ja and ( S )- 3ga could go through a thermal [2+2] reaction [34] , [35] to construct the tricyclic product 13ja containing two highly strained four-membered rings and bicyclic product ( S )- 13ga containing one highly strained four-membered ring in very high yields. (3) In addition, the hydrogenation or semi-hydrogenation of the carbon–carbon triple bond in ( S )- 3gj afforded saturated ( S )- 14 under 15 mol% of Pd/C catalyst or ( S,Z )- 15 with a Z -double bond under 10 mol% of the Lindlar catalyst, respectively [36] , [37] . 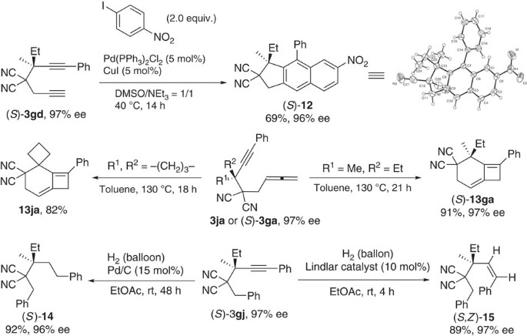Figure 5: The synthetic applications. Several molecules with two continuous all-carbon quaternary carbons centres were afforded. Figure 5: The synthetic applications. Several molecules with two continuous all-carbon quaternary carbons centres were afforded. Full size image In conclusion, we have developed a new concept of a palladium-catalysed propargylation of functionalized tri-substituted carbon nucleophiles with tertiary propargylic carbonates, which provides a very practical and useful method to construct a C–C bond between two tert-carbon atoms forming different 1,6-allenyne, 1,6-diyne, 1,6-enyne and 1,6-arenyne derivatives, which are important types of versatile compounds in organic chemistry-related disciplines. Moreover, no racemization occurred to the central chirality in the tertiary propargylic carbonates, which makes enantioselective synthesis of such molecules possible. Due to the presence of the triple bond and the demonstrated scope of the substrates, this reaction expands the scope of the existing methodologies for the construction of two vicinal all-carbon quaternary centres. Further studies on expanding the scope of the reaction, the mechanism, synthetic applications and development of enantioselective version of this reaction are being actively pursued in our laboratory. Materials DMSO was stirred with CaH 2 for 12 h at 80 °C and distilled in vacuo before use. Pd(OAc) 2 was purchased from Acros. Dppf was purchased from Energy Chemical. K 2 CO 3 was purchased from Sinopharm Chemical Reagent Co., Ltd. Pd/C was purchased from Alfa Aesar. Lindlar catalyst was purchased from J&K. Other commercially available chemicals were purchased and used without additional purification unless noted otherwise. General spectroscopic methods 1 H nuclear magnetic resonance (NMR) spectra were recorded on a Bruker-300 MHz spectrometer and 13 C NMR spectra were recorded at 75 MHz. All 1 H NMR experiments were measured with tetramethylsilane (0 p.p.m.) or the signal of residual CHCl 3 (7.26 p.p.m.) in CDCl 3 as the internal reference; 13 C NMR experiments were measured relative to the signal of CDCl 3 (77.0 p.p.m.). Infrared spectra were recorded from films of pure samples on sodium chloride plates for liquid samples or in the form of KBr discs for solid samples. Mass and HRMS spectra were carried out in EI mode. Elemental analysis was carried out by Elementar Vario MICRO cube. Thin-layer chromatography was performed on pre-coated glass-back plates and visualized with UV light at 254 nm. Flash column chromatography was performed on silica gel. 1 H NMR, 13 C NMR and HPLC spectra (for chiral compounds) are supplied for all compounds (see Supplementary Figs 1–137 ). See Supplementary Methods for the characterization data of compounds not listed in this part. Synthesis of 3aa To a flame-dried Schlenk tube containing K 2 CO 3 (414.2 mg, 3.0 mmol) were added Pd(OAc) 2 (11.4 mg, 0.05 mmol), dppf (33.4 mg, 0.06 mmol), 1a (217.5 mg, 1.0 mmol)/DMSO (8.0 ml) and 2a (178.0 mg, 1.5 mmol)/DMSO (2.0 ml) sequentially under nitrogen atmosphere. The reaction was complete after being stirred at 30 °C for 11 h as monitored by TLC (eluent: petroleum ether/ethyl acetate=20/1). After cooling to room temperature (rt), the resulting mixture was quenched with an aqueous solution of diluted hydrochloric acid ( v/v =10%, prepared via diluting commercially available concentrated hydrochloric acid with water according to the volume ratio; 10 ml) slowly and extracted with ethyl ether (30 ml × 3). The combined organic layer was washed with water and brine, and dried over anhydrous Na 2 SO 4 . After filtration and evaporation of the solvent, chromatography on silica gel (eluent: petroleum ether/ethyl acetate=20/1) afforded 3aa (226.4 mg, 89%) as a liquid: 1 H NMR (300 MHz, CDCl 3 ) δ 7.46–7.38 (m, 2H, ArH), 7.36–7.25 (m, 3H, ArH), 5.40–5.28 (m, 1H, CH=), 4.95 (dt, J 1 =6.7 Hz, J 2 =2.4 Hz, 2H, =CH 2 ), 2.82 (dt, J 1 =7.6 Hz, J 2 =2.3 Hz, 2H, CH 2 ), 1.63 (s, 6H, Me × 2); 13 C NMR (75 MHz, CDCl 3 ) δ 210.5, 131.6, 128.7, 128.2, 121.5, 113.9, 87.9, 85.9, 83.0, 77.1, 48.7, 39.4, 33.7, 25.7; IR (neat, cm −1 ) 3,063, 2,985, 2,942, 2,869, 2,245, 2,221, 1,956, 1,598, 1,491, 1,470, 1,459, 1,443, 1,393, 1,373, 1,291, 1,252, 1,161, 1,091, 1,071, 1,028; MS (EI): m/z (%) 260 (M + , 100); HRMS calcd. for C 18 H 16 N 2 (M + ): 260.1313; found: 260.1310. Synthesis of ( S )-3ga Following the procedure for the synthesis of 3aa , the reaction of K 2 CO 3 (413.7 mg, 3.0 mmol), Pd(OAc) 2 (11.4 mg, 0.05 mmol), dppf (33.3 mg, 0.06 mmol), ( S )- 1g (97% ee, 233.2 mg, 1.0 mmol)/DMSO (8.0 ml) and 2a (177.5 mg, 1.5 mmol)/DMSO (2.0 ml) at 30 °C for 12 h afforded ( S )- 3ga (217.5 mg, 79%) as a liquid (eluent: petroleum ether/ethyl acetate=20/1): 97% ee (HPLC conditions: Chiralcel IC column, hexane/ i -PrOH=200/1, 0.6 ml/min, λ =214 nm, t R (major)=35.3 min, t R (minor)=37.8 min); [ α ] D 20 =+32.2 ( c =1.055, CHCl 3 ); 1 H NMR (300 MHz, CDCl 3 ) δ 7.49–7.39 (m, 2H, ArH), 7.38–7.26 (m, 3H, ArH), 5.41–5.28 (m, 1H, =CH), 4.95 (dt, J 1 =6.5 Hz, J 2 =2.3 Hz, 2H, =CH 2 ), 2.94–2.75 (m, 2H, CH 2 ), 2.11–1.95 (m, 1H, one proton of CH 2 ), 1.86–1.71 (m, 1H, one proton of CH 2 ), 1.56 (s, 3H, Me), 1.21 (t, J =7.4 Hz, 3H, Me); 13 C NMR (75 MHz, CDCl 3 ) δ 210.7, 131.7, 128.8, 128.3, 121.7, 114.1, 87.3, 86.7, 83.1, 77.1, 49.3, 44.1, 33.7, 30.7, 21.7, 9.5; IR (neat, cm −1 ) 3,062, 2,978, 2,941, 2,883, 2,247, 2,228, 1,956, 1,598, 1,491, 1,461, 1,443, 1,386, 1,321, 1,250, 1,131, 1,091, 1,070; MS (EI): m/z (%) 274 (M + , 100); HRMS calcd. for C 19 H 18 N 2 (M + ): 274.1470; Found: 274.1469. Synthesis of ( S )-12 To a flame-dried Schlenk tube were added Pd(PPh 3 ) 2 Cl 2 (17.6 mg, 0.025 mmol), CuI (4.9 mg, 0.025 mmol), 1-iodo-4-nitrobenzene (249.3 mg, 1.0 mmol), ( S )- 3gd (97% ee, 130.2 mg, 0.5 mmol)/DMSO (2.0 ml) and NEt 3 (2.0 ml) sequentially under nitrogen atmosphere. The reaction was complete after being stirred at 40 °C for 14 h as monitored by TLC (eluent: petroleum ether/ethyl acetate=10/1). After cooling to rt, the resulting mixture was diluted with ethyl acetate (30 ml) and washed with water (20 ml). The organic layer was separated and the aqueous layer was extracted with ethyl acetate (20 ml). The combined organic layer was washed with brine and dried over anhydrous Na 2 SO 4 . After filtration and evaporation, the residue was purified by chromatography (eluent: petroleum ether/ethyl acetate/dichloromethane=10/1/1) on silica gel to afford ( S )- 12 (129.5 mg, 69%) as a solid: 96% ee (HPLC conditions: Chiralcel OD-H column, hexane/ i -PrOH=80/20, 1.0 ml min −1 , λ =214 nm, t R (major)=9.5 min, t R (minor)=10.3 min); [ α ] D 20 =−33.9 ( c =0.975, CHCl 3 ); m.p. 205–206 °C ( n -hexane/DCM); 1 H NMR (300 MHz, CDCl 3 ) δ 8.26–8.18 (m, 2H, ArH), 8.00–7.93 (m, 1H, ArH), 7.90 (s, 1H, ArH), 7.62–7.49 (m, 3H, ArH), 7.34–7.22 (m, 2H, ArH), 3.93 (dd, J 1 =16.4 Hz, J 2 =1.1 Hz, 1H, one proton of CH 2 ), 3.84 (dd, J 1 =16.5 Hz, J 2 =1.2 Hz, 1H, one proton of CH 2 ), 1.95–1.78 (m, 1H, one proton of CH 2 ), 1.58–1.39 (m, 1H, one proton of CH 2 ), 1.42 (s, 3H, Me), 0.98 (t, J =7.5 Hz, 3H, Me); 13 C NMR (75 MHz, CDCl 3 ) δ 145.7, 141.9, 139.2, 138.0, 135.4, 135.3, 133.1, 130.4, 130.1, 129.1, 128.9, 128.50, 128.46, 123.7, 123.1, 119.9, 115.3, 114.8, 57.3, 44.8, 41.6, 32.3, 22.9, 9.2; IR (KBr, cm −1 ) 3,078, 3,057, 2,978, 2,931, 2,883, 2,249, 1,628, 1,610, 1,584, 1,531, 1,490, 1,460, 1,442, 1,391, 1,377, 1,339, 1,287, 1,266, 1,218, 1,090, 1,054, 1,028; MS (EI): m/z (%) 381 (M + , 51.55), 352 (100); anal. calcd. for C 24 H 19 N 3 O 2 (%): C 75.57, H 5.02, N 11.02; found: C 75.60, H 5.05, N 11.19. Synthesis of 13ja To a flame-dried Schlenk tube was added 3ja (273.2 mg, 1.0 mmol)/toluene (10 ml) under nitrogen atmosphere. The reaction was complete after being stirred at 130 °C for 18 h as monitored by TLC (eluent: petroleum ether/ethyl acetate=20/1). After cooling to rt and evaporation of the solvent, the residue was purified by chromatography (eluent: petroleum ether/ethyl acetate/dichloromethane=20/1/1) on silica gel to afford 13ja (223.1 mg, 82%) as a solid: m.p. 133–135 °C ( n -hexane/DCM); 1 H NMR (300 MHz, CDCl 3 ) δ 7.54–7.29 (m, 5H, ArH), 5.17 (t, J =3.9 Hz, 1H, =CH), 3.32 (s, 2H, CH 2 ), 2.86 (d, J =3.9 Hz, 2H, CH 2 ), 2.80–2.43 (m, 4H, CH 2 × 2), 2.40–2.21 (m, 2H, CH 2 ); 13 C NMR (75 MHz, CDCl 3 ) δ 142.1, 139.1, 138.5, 133.4, 128.7, 128.6, 127.2, 115.2, 102.0, 44.6, 42.4, 35.9, 31.9, 28.6, 14.0; IR (KBr, cm −1 ) 3,056, 2,991, 2,941, 2,914, 2,247, 1,754, 1,595, 1,490, 1,445, 1,435, 1,353, 1,321, 1,246, 1,180, 1,157, 1,097, 1,033; MS (EI): m/z (%) 272 (M + , 39.83), 244 (100); anal. calcd. for C 19 H 16 N 2 (%): C 83.79, H 5.92, N 10.29; found: C 83.58, H 5.85, N 10.25. Synthesis of 14 To a dry Schlenk tube were added Pd/C (dry, w/w (Pd)=10%, 32.2 mg, 0.03 mmol) and 3gj (63.0 mg, 0.2 mmol)/EtOAc (4 ml) sequentially. The resulting mixture was frozen with a liquid nitrogen bath, degassed and refilled with H 2 for three times. Then the reaction was allowed to stir at rt with a H 2 balloon. After 48 h, the reaction was completed as monitored by TLC (petroleum ether/ethyl acetate=20/1). The mixture was filtrated through a short column of silica gel with EtOAc (20 ml × 3). After evaporation, the residue was purified by chromatography (eluent: petroleum ether/ethyl acetate=15/1) on silica gel to afford 14 (57.1 mg, 89%) as a solid: m.p. 112–113 °C (hexane/DCM); 1 H NMR (300 MHz, CDCl 3 ): δ 7.50–7.15 (m, 10H, ArH), 3.13 (s, 2H, CH 2 ), 2.86–2.64 (m, 2H, CH 2 ), 2.12–1.70 (m, 4H, CH 2 × 2), 1.34 (s, 3H, Me), 1.14 (t, J =7.4 Hz, 3H, Me); 13 C NMR (75 MHz, CDCl 3 ) δ 141.2, 132.7, 130.5, 128.7, 128.63, 128.58, 128.2, 126.3, 115.0, 49.7, 43.5, 38.4, 38.0, 30.8, 29.0, 21.5, 9.0; IR (KBr, cm −1 ) 3,087, 3,066, 3,024, 2,975, 2,949, 2,881, 2,239, 1,599, 1,498, 1,472, 1,455, 1,435, 1,386, 1,239, 1,090, 1,031, 1,010; MS (EI): m/z (%) 316 (M + , 2.17), 91 (100); anal. calcd. for C 22 H 24 N 2 (%): C 83.50, H 7.64, N 8.85; found: C 83.41, H 7.72, N 8.75. Synthesis of ( S , Z )-15 Following procedure for the synthesis of 14 , the reaction of lindlar catalyst (palladium on calcium carbonate, w/w (Pd)=5%, poisoned with lead acetate, 42.5 mg, 0.02 mmol), ( S )- 3gj (62.0 mg. 0.2 mmol) and H 2 in EtOAc (4.0 ml) at rt for 4 h afforded ( S,Z )- 15 (55.7 mg, 89%) as a solid (eluent: petroleum ether/ethyl acetate=30/1): 97% ee (high-performance liquid chromatography (HPLC) conditions: Chiralcel AD-H column, hexane/ i -PrOH=200/1, 0.6 ml min −1 , λ =214 nm, t R (minor)=35.5 min, t R (major)=41.2 min); [ α ] D 20 =+142.7 ( c =0.96, CHCl 3 ); m.p. 112–113 °C (hexane/dichloromethane (DCM)); 1 H NMR (300 MHz, CDCl 3 ): δ 7.47–7.23 (m, 8H, ArH), 7.22–7.14 (m, 2H, ArH), 7.09 (d, J =12.9 Hz, 1H, CH=), 5.62 (d, J =12.9 Hz, 1H, CH=), 3.22 (d, J =13.2 Hz, 1H, one proton of CH 2 ), 3.11 (d, J =13.2 Hz, 1H, one proton of CH 2 ), 2.04–1.88 (m, 1H, one proton of CH 2 ), 1.81–1.67 (m, 1H, one proton of CH 2 ), 1.02 (t, J =7.4 Hz, 3H, Me), 0.98 (s, 3H, Me); 13 C NMR (75 MHz, CDCl 3 ) δ 137.4, 135.9, 132.8, 130.4, 130.1, 128.8, 128.5, 128.0, 127.8, 127.1, 114.60, 114.56, 51.1, 49.4, 38.8, 31.8, 18.8, 9.0; IR (KBr, cm −1 ) 3,062, 3,033, 2,974, 2,941, 2,881, 2,242, 1,599, 1,492, 1,456, 1,442, 1,388, 1,124, 1,090, 1,071, 1,025; MS (EI): m/z (%) 314 (M + , 0.13), 159 (100); anal. calcd. for C 22 H 22 N 2 (%): C 84.04, H 7.05, N 8.91; found: C 83.95, H 7.11, N 8.78. Data availability The authors declare that all the data supporting the findings of this study are available within the article and its Supplementary Information files. How to cite this article: Huang, X. et al . Palladium-catalysed formation of vicinal all-carbon quaternary centres via propargylation. Nat. Commun. 7:12382 doi: 10.1038/ncomms12382 (2016).